Designing attractive models via automated identification of chaotic and oscillatory dynamical regimes Chaos and oscillations continue to capture the interest of both the scientific and public domains. Yet despite the importance of these qualitative features, most attempts at constructing mathematical models of such phenomena have taken an indirect, quantitative approach, for example, by fitting models to a finite number of data points. Here we develop a qualitative inference framework that allows us to both reverse-engineer and design systems exhibiting these and other dynamical behaviours by directly specifying the desired characteristics of the underlying dynamical attractor. This change in perspective from quantitative to qualitative dynamics, provides fundamental and new insights into the properties of dynamical systems. Mathematical modelling requires a combination of experimentation, domain knowledge and, at times, a measure of luck. Beyond the intrinsic challenges of describing complex and complicated phenomena, the difficulty resides at a very fundamental level with the diversity of models that could explain a given set of observations. This is a manifestation of the so-called inverse problem [1] , which is encountered whenever we aim to reconstruct a model of the process from which data have been generated. Exploring the potential space of solutions computationally can be prohibitively expensive and will generally require sophisticated numerical approaches or search heuristics, as well as expert guidance and manual interventions. Parameter estimation [2] , model inference [3] and model selection [4] , [5] all address aspects of this problem. The inverse problem also applies in a different context: the design of systems with specified or desired outputs. Here again we have a multitude of different models—or, for sufficiently complicated models, a potentially vast range of parameters—that fulfil a given set of design objectives. Therefore, system design can be fraught with the same challenges as statistical inference or reverse-engineering tasks: in the former case, we want to learn the existing structure and properties of a system that has produced certain types of data, whereas in the latter we want to design constructible systems that will reliably and robustly exhibit certain types of behaviour. These challenges are often further exacerbated by unsuitable or insufficient encoding of the behaviour that we observe (in natural systems) or would like to see (in designed systems). For example, if we aim to estimate parameters describing an oscillating system from a series of observations, it is possible to get good and even globally optimal fits to the data, without finding a qualitatively acceptable solution. Various methods of qualitative inference have been developed to address this issue; the topology of bifurcation diagrams [6] , [7] , local stability properties of dynamically invariant sets [8] , [9] , symbolic sequences of chaotic systems [10] and temporal logic constraints [11] , [12] have variously been used to drive parameter searches, or for model checking. However, these methods are either limited in the complexity of behaviour they can detect, or by conditioning on surrogate data (for example, forcing solutions through a small number of points), they suffer in the same way as quantitative approaches. The method proposed here extends the scope of the promising, but underdeveloped, class of qualitative parameter estimation algorithms [13] , allowing detection and control of the most complex and elusive dynamical behaviours, such as oscillations, chaos and hyperchaos. We consider models of the general form where y ( t ) denotes the n -dimensional state of the system at time t ; f is the gradient field characterized by a parameter vector; θ , and y 0 = y (0) are the initial conditions, which may also be unknown. Coaxing the solutions of such systems into exhibiting a desired dynamical behaviour is reliant on the ability to, first, encode the behaviour sufficiently as constraints on a set of model properties that may be conveniently evaluated, and second, to identify regions in parameter space for which these constraints are satisfied. Here we meet these challenges using a combination of statistical and dynamical systems techniques. In particular, we pose the problem within a state–space framework, where the observation function corresponds to evaluating the type of attractor exhibited by the model with given parameters and initial conditions. We then exploit the flexibility and efficiency of the unscented Kalman filter (UKF) to systematically move in parameter space until the desired or expected dynamical behaviour is exhibited. 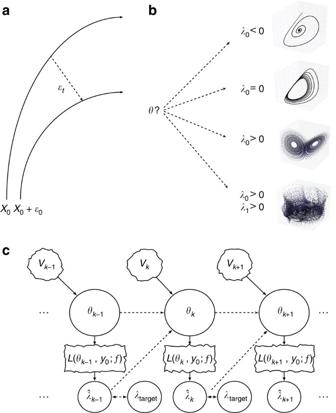Figure 1: Encoding and inferring the desired dynamics. (a) LEs,λ0, ...λn, characterize the contraction/expansion of an initially small perturbation,ɛ0, to the system. (b) The leading LE determines the principal dynamics and characteristics of the attractor of a dynamical system. Forλ0<0, the attractor will be a stable fixed point; stable oscillating solutions will be obtained, ifλ0=0; forλ0>0 we observe chaos and the system will exhibit a so-called strange attractor; if more than one LE is positive, then we speak of hyperchaos and the attractor will exhibit behaviour with similar statistical properties to white noise. (c) Key steps in the UKF for qualitative inference. At thekthiteration, the current prior parameter distribution is formed by perturbing the previous posterior,θk, with the process noisevk. The distribution of LEs for the modelfinduced by the prior parameter distribution is calculated via the LE estimation routine L and the unscented transform. Comparing the mean LE,, to the target LE,λtarget, the prior parameters are updated using the UKF update equations. As the filter proceeds, parameters are found that locally minimise the sum of squared error between target and estimated LEs. The approach, outlined in Figure 1 and developed fully in the Methods and Supplementary Information , is demonstrated below within different contexts, covering some classical dynamical model systems and electronic circuits that exhibit oscillations, chaos and hyperchaos, and a biological regulatory system that exhibits oscillatory behaviour. Figure 1: Encoding and inferring the desired dynamics. ( a ) LEs, λ 0 , ... λ n , characterize the contraction/expansion of an initially small perturbation, ɛ 0 , to the system. ( b ) The leading LE determines the principal dynamics and characteristics of the attractor of a dynamical system. For λ 0 <0, the attractor will be a stable fixed point; stable oscillating solutions will be obtained, if λ 0 =0; for λ 0 >0 we observe chaos and the system will exhibit a so-called strange attractor; if more than one LE is positive, then we speak of hyperchaos and the attractor will exhibit behaviour with similar statistical properties to white noise. ( c ) Key steps in the UKF for qualitative inference. At the k th iteration, the current prior parameter distribution is formed by perturbing the previous posterior, θ k , with the process noise v k . The distribution of LEs for the model f induced by the prior parameter distribution is calculated via the LE estimation routine L and the unscented transform. Comparing the mean LE, , to the target LE, λ target , the prior parameters are updated using the UKF update equations. As the filter proceeds, parameters are found that locally minimise the sum of squared error between target and estimated LEs. Full size image Oscillations and chaos in electronic circuits The elimination of chaos from a system, or conversely its 'chaotification', have potential applications to biological, medical, information processing and other technological systems [14] . Here we use a simple electric circuit [15] (shown in Fig. 2a ), to illustrate how our method can be used to tune the system parameters such that the dynamics are driven into and out of chaos. The circuit model includes a parameter a , representing the scaled resistance of a variable resistor, R 2 , which we make the lone subject of the inference. In turn, we start the system in an oscillatory regime and tune the parameter according to the posterior predictions at each step of the UKF, until we enter a chaotic regime, and vice versa (see Fig. 2b ). The two desired behaviours are encoded as constraints only on the target maximal Lyapunov exponent (LE), specifying, λ 1 =0, for oscillations, and, λ 1 = d > δ tol for chaos, where δ tol is taken larger-than-the-expected error in the LE estimation procedure, as discussed in the Supplementary Information . 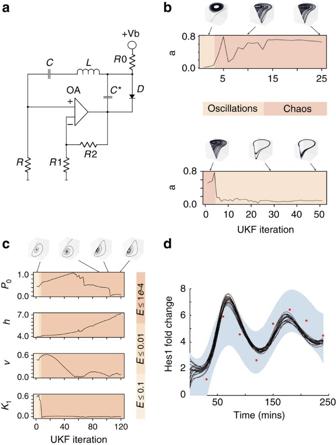Figure 2: Detecting and controlling chaos and oscillations. Plots show the estimated parameters at successive iterations of the UKF. Snapshots of the developing attractor are shown above the plots. The sum of squared error (E) is indicated for different sections of the parameter trajectories. (a) Diagram of the circuit investigated. (b) The filter is able to drive the electric circuit between oscillations and chaos in less than 10 iterations. (c) Parameter trajectories for a simple model of the Hes1 regulatory system that yield oscillations. Several regions in parameter space can be identified that exhibit oscillatory behaviour. (d) Examples of trajectories generated from a region in parameter space that was found using our approach. Here we used the qualitative inference procedure to elicit a prior to be used for parameter inference. Trajectories were sampled from the prior. Data are indicated by red circles and represent fold change in Hes1 mRNA; the blue strips indicate the confidence intervals obtained using Gaussian process regression, in which standard Gaussian noise is assumed, with maximum marginal likelihood estimates for the other hyperparameters21. Figure 2: Detecting and controlling chaos and oscillations. Plots show the estimated parameters at successive iterations of the UKF. Snapshots of the developing attractor are shown above the plots. The sum of squared error ( E ) is indicated for different sections of the parameter trajectories. ( a ) Diagram of the circuit investigated. ( b ) The filter is able to drive the electric circuit between oscillations and chaos in less than 10 iterations. ( c ) Parameter trajectories for a simple model of the Hes1 regulatory system that yield oscillations. Several regions in parameter space can be identified that exhibit oscillatory behaviour. ( d ) Examples of trajectories generated from a region in parameter space that was found using our approach. Here we used the qualitative inference procedure to elicit a prior to be used for parameter inference. Trajectories were sampled from the prior. Data are indicated by red circles and represent fold change in Hes1 mRNA; the blue strips indicate the confidence intervals obtained using Gaussian process regression, in which standard Gaussian noise is assumed, with maximum marginal likelihood estimates for the other hyperparameters [21] . Full size image For systems of this size, the qualitative dynamical regimes can be explored exhaustively and in short time (finding the desired behaviour takes minutes even for moderate sized systems). Detecting oscillations in immune signalling Oscillations appear to be ubiquitous in nature, yet, for reasons noted above, they often remain elusive to quantitatively driven parameter inference techniques. Here we consider a dynamical system describing the expression levels of the transcription factor Hes1, which is involved in regulating the segmentation of vertebrate embryos [16] . Oscillations of Hes1 expression levels have been observed in vitro in mouse cell lines, and reproduced using various modelling approaches, including continuous deterministic delay [16] , [17] and discrete stochastic delay models [18] . We investigate a simple three-component ordinary differential equation (ODE) model of the regulatory dynamics with mRNA transcription modelled by a Hill function, where state variables M , P 1 and P 2 , are the molecular concentrations of Hes1 mRNA, cytoplasmic and nuclear proteins, respectively. The parameter k deg is the Hes1 protein degradation rate that we assume to be the same for both cytoplasmic and nuclear proteins; k 1 is the rate of transport of Hes1 protein into the nucleus; P 0 is the amount of Hes1 protein in the nucleus, when the rate of transcription of Hes1 mRNA is at half its maximal value; ν is the rate of translation of Hes1 mRNA, and h is the Hill coefficient. For the inference we take, k deg , to be the experimentally determined value of 0.03 min −1 (ref. 19 ). In Figure 2c, we show the results for the inference using our algorithm on the model shown above. Note that the value inferred for parameter k 1 , is significantly lower than the range of values investigated for the continuous deterministic delay model of Momiji and Monk [17] . Interestingly, repeating the inference with different initial parameter sets leads to similar values of k 1 ( k 1 <0.01), but to a broad range of values for the other parameters, all of which result in oscillatory behaviour. Our qualitative inference thus suggests that oscillations of Hes1 protein and mRNA levels are strongly dependent on maintaining a low rate of transport of Hes1 protein into the nucleus, and that the dependence on other system parameters is less strong. As 1/ k 1 is the expected time Hes1 spends in the cytoplasm, this corresponds to the delay that had previously been posited to be necessary for such oscillations to occur [17] . Our approach readily identifies a parameter regime exhibiting oscillatory dynamics without explicitly requiring (discrete) time delays. Next, we used the qualitative inference result as the basis to estimate the model parameters from the Hes1 data described below. An approximate Bayesian computation algorithm (ABC SMC [20] ), capable of sampling from non-Gaussian and multimodal posteriors, was employed and Figure 2d shows the fits of simulated trajectories for 20 parameters drawn randomly from the resulting posterior distribution; these are in good agreement with the confidence intervals (the blue bands in Fig. 2d ), which can be obtained from the time-course data via a Bayesian nonparametric method [21] . It is worth noting that using the UKF alone, we could in principle consider the LEs and data together to infer parameters that are both qualitatively and quantitatively acceptable. However, by splitting the inference, we take advantage of the strengths of each algorithm within the Bayesian framework; first we exploit the efficiency of the UKF to work with a sophisticated encoding of the desired behaviour that is computationally expensive to calculate; subsequently we use this qualitative information to construct suitable priors for an ABC method capable of dealing with non-Gaussian posteriors. Designing attractors Although the maximal LE alone is sufficient to encode fixed points, limit cycles and strange attractors, we may include extra target exponents to design the complete Lyapunov spectrum ( Fig. 3a ), design the (Kaplan–Yorke) fractal dimension [22] , where k is the largest integer for which of a system's attractor ( Fig. 3b ), or drive models to behave hyper-chaotically ( Fig. 3c ). 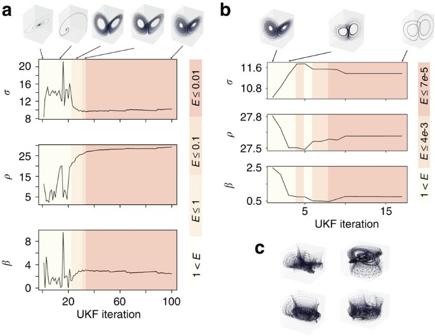Figure 3: Designing attractive models. (a) Inferring a complete spectrum. After only 22 iterations, the characteristic 'butterfly' strange attractor emerges. The final parameters and LEs areσ=10.2,ρ=29.2,β=2.45 and (0.899, 2.74×10−4, −14.6). (b) A function of the LEs, the Kaplan–Yorke fractal dimension may also be used to specify the desired attractor. Here parameters for a target dimension of 1 are found for the Lorenz system within 20 iterations, giving rise to a limit cycle as required by the theory. (c) Three-dimensional projections of the hyperchaotic system with parameter vector (a,b,c,d,e,f)=(49.98, 35.86, 30.5, 1.35, 36.6, 33.8) and corresponding LEs (31.8, 16.8, −19.1, −71.4). Within a few iterations, our algorithm was able to drive the system towards an attractor characterized by LEs twice the size of any that had previously been reported. Figure 3: Designing attractive models. ( a ) Inferring a complete spectrum. After only 22 iterations, the characteristic 'butterfly' strange attractor emerges. The final parameters and LEs are σ =10.2, ρ =29.2, β =2.45 and (0.899, 2.74×10 −4 , −14.6). ( b ) A function of the LEs, the Kaplan–Yorke fractal dimension may also be used to specify the desired attractor. Here parameters for a target dimension of 1 are found for the Lorenz system within 20 iterations, giving rise to a limit cycle as required by the theory. ( c ) Three-dimensional projections of the hyperchaotic system with parameter vector ( a , b , c , d , e , f )=(49.98, 35.86, 30.5, 1.35, 36.6, 33.8) and corresponding LEs (31.8, 16.8, −19.1, −71.4). Within a few iterations, our algorithm was able to drive the system towards an attractor characterized by LEs twice the size of any that had previously been reported. Full size image The first two of these applications are illustrated with the Lorenz system [23] which has become a canonical example of how sensitivity to initial conditions can give rise to unpredictable behaviour. The model is known to exhibit a chaotic regime with LEs, Λ =(0.906, 0, −14.57), for parameter vector ( σ , ρ , β )=(10, 28, 8/3). Here we infer back these parameters, starting with different prior means, by setting our target Lyapunov spectrum to Λ . If we restrict the parameter search to the region [0, 30] 3 , as described in the Supplementary Information , we are able to do this reliably from random starting positions. The parameter trajectories and evolving attractor of a representative run of the inference algorithm is shown in Figure 3a , where the sum of squared error between estimated and target LEs is less than 8×10 −5 after the 100th iteration. Without constraints on the parameters, the inference algorithm converges to different parameter combinations that display indistinguishable LEs. This allows us to assess (for example) the robustness of chaotic dynamics by mapping systematically the regions of parameter space that yield similar LEs. Figure 3b shows how the fractal dimension—a function of the LEs—may also be tuned (in this example, halved). Although computational difficulties have in the past precluded such investigations, our approach allows us to map attractor structures (and the range of parameters giving rise to similar attractors) very efficiently. For the third application of driving a system into hyper-chaos, we investigate a four-dimensional system with six parameters, whose significance lies in having two very large LEs ( λ 1 ∈ [10.7741, 12.9798] and λ 2 ∈ [0.4145, 2.6669]) over a broad parameter range [24] . The resulting highly complex deterministic dynamics share statistical properties with white noise, making it attractive for engineering applications such as communication encryption and random number generation. By setting large target values of λ 1 and λ 2 , we use our method to obtain parameters for which the system displays LEs that are over two times bigger than previously found for the system. Figure 3c shows the three-dimensional projections of the resulting hyper-chaotic attractor. These are, of course, toy applications, but they demonstrate the flexibility and potential uses of this approach: we can really start to explore qualitative behaviour in a numerically efficient and speedy manner. For example, it becomes possible to map (or design) the qualitative characteristics of complex systems and to test robustness of qualitative system features systematically. We have demonstrated that it is possible to use statistical inference techniques to condition dynamical systems on observed (biological oscillations in Hes1) or desired qualitative characteristics (oscillations, chaos and hyper-chaos in natural and engineered systems). This provides us with unprecedented ability to probe the workings of dynamical systems. Here we have only used the approach for inference and design of the attractors of dynamical systems, as encoded by their LEs. This, however, has already been enough to show that it is not necessary to impose discrete time delays to explain the oscillations in the Hes1 system [16] , [17] , [18] . A focus on qualitative features has several advantages: first, it is notoriously difficult, for example, to ensure that parameter inference preferentially (let alone exclusively) explores regions in parameter space that correspond to the correct qualitative behaviour such as oscillations. This is the case for optimization as well as the more sophisticated estimation procedures. Arguably, however, solutions that display the correct qualitative behaviour are more interesting than those that locally minimize some cost-function in light of some limited data. Obviously, in a design setting, ensuring the correct qualitative behaviour is equally important. Second, the numerical performance of the current approach allows us to study fundamental aspects related to the robustness of qualitative behaviour. This allows us, for the first time, to ascertain how likely a system is to produce a given Lyapunov spectrum (and hence attractor dimension) for different parameter values, θ . Our approach, coupled with means of covering large-dimensional parameter spaces, such as Latin-hypercube or Sobol sampling [25] , allows us to explore such qualitative robustness. Or more specifically, we can map out boundaries separating areas in phase space with different qualitative types of behaviour. We can also drive systems into regions with LEs of magnitudes not previously observed. The last aspect will have particular appeal to information and communication scientists as such hyper-chaos shares important properties with white noise and potential applications in cryptography and coding theory abound [26] . Finally, our approach can also be used to condition dynamical systems on all manner of observed or desired qualitative dynamics, such as threshold behaviour, bifurcations, robustness, temporal ordering and so on. To rule out that a mathematical model can exhibit a certain dynamical behaviour will, however, require exhaustive numerical sampling of the parameter space; but coupled to ideas from probabilistic computing [27] ; our procedure lends itself to such investigations. Both for inference and design problems, we foresee vast scope for applying this type of qualitative inference-based modelling. There is still a lack of understanding about the interplay between qualitative and quantitative features of dynamical systems [28] ; this becomes more pressing to address as the systems we are considering become more complicated and the data collected more detailed. Flexibility in parameter estimation—whether based on qualitative or quantitative system features—will be an important feature for the analysis of such system, as well as the design of synthetic systems in engineering and synthetic biology. Encoding dynamics through Lyapunov exponents Consider a continuous time dynamical system—similar results hold for the discrete case—described by, where f is an n -dimensional gradient field. To study the sensitivity of f to initial conditions, we consider the evolution of an initially orthonormal axes of n vectors, { ɛ 1 , ɛ 2 , ..., ɛ n }, in the tangent space at y 0 . At time t , each ɛ i satisfies the linear equation, where Df ( y t ) is the Jacobian of f evaluated along the orbit y t . Equations (5) and (6) describe the expansion/contraction of an n -dimensional ellipsoid in the tangent space at y t , and we denote the average exponential rate of growth over all t of the i th principal axis of the ellipsoid as λ i . The quantities, λ 1 ≥ λ 2 ≥ ... ≥ λ n , are called the global LEs of f . In particular, the sign of the maximal LE, λ 1 , determines the fate of almost all small perturbations to the system's state, and consequently, the nature of the underlying dynamical attractor. For λ 1 <0, all small perturbations die out and trajectories that start sufficiently close to each other converge to the same stable fixed point in state-space; for λ 1 =0, initially close orbits remain close but distinct, corresponding to oscillatory dynamics on a limit-cycle or torus (for tori, at least one other exponent must be zero); and finally for λ 1 >0, small perturbations grow exponentially, and the system evolves chaotically within the folded space of a so-called 'strange attractor' (for two or more positive definite LEs, we speak of 'hyperchaos'). In general, nonlinear system equations and the asymptotic nature of the LEs precludes any analytic evaluation. Instead, various methods of numerical approximation of these quantities, both directly from ODE models and from time-series data [29] , [30] , [31] have been developed. In this paper, Lyapunov spectra are calculated using a Python implementation of a method proposed by Benettin et al . [32] and Shimada and Nagashima [33] (outlined in the Supplementary Information ) for inference of LEs when the differential equations are known. Lyapunov spectrum driven parameter estimation Unlike in the case for linear systems, where identifying suitable parameters that produce observed or desired dynamics is trivial, inference for highly nonlinear systems is far from straightforward. Indeed, exact inferences are prohibitively expensive for even small systems, and so a host of different approximation methods have been proposed [20] , [34] , [35] . In our case, two further complications arise from using LEs to encode the desired behaviour. First, the form of the mapping between model parameters and LEs is not closed, making methods that rely on an approximation of the estimation routine or its derivatives, such as the extended Kalman filter, difficult to apply. Second, LEs are significantly more expensive to compute than more traditional cost functions, ruling out the use of approaches such as particle filtering or sequential Monte-Carlo methods that require extensive sampling of regions of parameter space and calculation of the corresponding LEs at each iteration. To overcome these challenges, we exploit the efficiency and flexibility of the UKF [36] , [37] , [38] , seeking here to infer the posterior distribution over parameters that give rise to the desired LEs. Typically, the UKF is applied for parameter estimation of a nonlinear mapping g (·) from a sequence of noisy measurements, y k , of the true states, x k , at discrete times k = t 1 , ..., t N . A dynamical state-space model is defined, where u k ∼ N (0, Q k ) represents the measurement noise, v k ∼ N (0, R k ) is the artificial process noise driving the system, and g (·) is the mapping for which parameters θ k are to be inferred. The UKF (described in full below) is then characterized by the iterative application of a two step, 'predict' and 'update', procedure. In the 'prediction step' the current parameter estimate is perturbed by the driving process noise v k forming a priori estimates (which are conditional on all but the current observation) for the parameter mean and covariance. These we denote as and , respectively. The 'update step' then updates the a priori statistics using the further measurement, y k , to form a posteriori estimates, and . After all observations have been processed, we arrive at the final parameter estimate, (with covariance ). A crucial step in the algorithm is the propagation of the a priori parameter distribution statistics through the model, g (·). Assuming linearity of this transformation, a closed form optimal filter may be derived (known as the Kalman filter). However, this assumption would make the algorithm inappropriate for use with the highly nonlinear systems and the choice of g (·) considered here. It is how the UKF copes with this challenge, namely its use of the 'unscented transform', that makes it particularly suitable for our method of qualitative feature-driven parameter estimation. The unscented transform is motivated by the idea that probability distributions are easier to approximate than highly nonlinear functions [39] . In contrast to the Extended Kalman filter where nonlinear state transition and observation functions are approximated by their linearized forms, the UKF defines a set, Θ k , of 'sigma-points'—deterministically sampled particles from the current posterior parameter distribution (given by and , that along with corresponding weights, , completely capture its mean and covariance. The sigma points can be propagated individually through the nonlinear observation function, and recombined to estimate the mean and covariance of the predicted observation, y k , to third-order accuracy in the Taylor expansion, using the equations given below. Under the approximate assumption of Gaussian prior and posterior distributions (higher order moments may be captured if desired at the cost of computational efficiency), the deterministic and minimal sampling scheme at the heart of the filter requires relatively few LE evaluations at each iteration (2 n p +1, where n p is the number of parameters to be inferred). Further, the function that is the subject of the inference may be highly-nonlinear and can take any parametric form, such as a feed-forward neural network [36] , or as in our case, a routine for estimating the LEs of a model with a given parameter set. With [ X ] i denoting the i th column of the matrix X , the UKF algorithm for parameter estimation is given by, Initialize: For each time point k = t 1 , ..., t N : Prediction step: Update step: where Various schemes for sigma-point selection exist including those for minimal set size, higher than third-order accuracy and (as defined and used in this study) guaranteed positive-definiteness of the parameter covariance matrices [39] , [40] , [41] , [42] , which is necessary for the square roots obtained by Cholesky decomposition when calculating the sigma points. The scaled sigma-point scheme thus proceeds as, where and parameters κ , α and β may be chosen to control the positive definiteness of covariance matrices, spread of the sigma-points, and error in the kurtosis, respectively. Our choices for the UKF parameter and noise covariances are discussed in the Supplementary Information . To apply to the UKF for qualitative inference, we amend the dynamical state-space model to, where L (·) maps parameters to the encoding of the dynamical behaviour (here a numerical routine to calculate the Lyapunov spectrum), λ target is a constant target vector of LEs, y 0 denotes the initial conditions, and f is the dynamical system under investigation (with unknown parameter vector θ , considered as a hidden state of the system and not subject to temporal dynamics). To see how equations (9) and (10) fit the state-space model format for UKF parameter estimation, it is helpful to consider the time series ( λ target , λ target , λ target , ...) as the 'observed' data from which we learn the parameters of the nonlinear mapping L (·). Our use of the UKF is characterized by a repeated comparison of the simulated dynamics for each sigma point to the same (as specified) desired dynamical behaviour. In this respect, we use the UKF as a smoother; there is no temporal ordering of the data supplied to the filter because all information about the observed (target) dynamics is given at each iteration. From an optimization viewpoint, the filter aims to minimize the prediction-error function, thus moving the parameters towards a set for which the system exhibits the desired dynamical regime. Hes 1 quantitative real-time PCR Dendritic cells were differentiated from bone marrow, as described previously [43] . Rat Jgd1/humanFc fusion protein (R&D Systems) or human IgG1 (Sigma Aldrich) (control samples) were immobilized onto tissue culture plates (10 μg ml −1 in PBS) overnight at 4 °C. Dendritic cells were spun onto the plate and cells were collected at the appropriate time. Total RNA was isolated using the Absolutely RNA micro prep kit (Stratagene). Complementary DNA was generated from 125 ng of total RNA using an archive kit (Applied Biosystems). 1 μl of cDNA was used with PCR Mastermix and TaqMan primer and probes (both Applied Biosystems) and analysed on an Applied Biosystems 7500 PCR system. Cycle thresholds were normalized to 18S and calibrated to a PBS-treated control sample for relative quantification. Computational implementation All routines were implemented in Python using LSODE for integrating differential equations. ABC inference was performed using the ABC-SysBio package [44] . Code is available from the authors on request. How to cite this article: Silk, D. et al . Designing attractive models via automated identification of chaotic and oscillatory dynamical regimes. Nat. Commun. 2:489 doi: 10.1038/ncomms1496 (2011).